Cooling and stabilization by collisions in a mixed ion–atom system In mixed systems of trapped ions and cold atoms, the ions and atoms can coexist at different temperatures. This is primarily due to their different trapping and cooling mechanisms. The key questions of how ions can cool collisionally with cold atoms and whether the combined system allows stable coexistence, need to be answered. Here we experimentally demonstrate that rubidium ions cool in contact with magneto-optically trapped rubidium atoms, contrary to the general experimental expectation of ion heating. The cooling process is explained theoretically and substantiated with numerical simulations, which include resonant charge exchange collisions. The mechanism of single collision swap cooling of ions with atoms is discussed. Finally, it is experimentally and numerically demonstrated that the combined ion–atom system is intrinsically stable, which is critical for future cold chemistry experiments with such systems. The cooling and trapping of particles facilitates their precise interrogation and manipulation. Cooling lowers the momentum spread of particles and allows the interparticle interactions to dominate the evolution of the system. Trapping spatially localizes the coordinates of particles, for convenient and extended study. The processes of cooling and trapping, although disparate in their nature, are both critical to studies with individual or collections of particles at low energies. Trapping and cooling of ions, and separately atoms, has been at the core of modern physics for decades. A mixed system of cooled and trapped atoms and trapped ions [1] , [2] , [3] , [4] , [5] , [6] paves the way for ion-assisted cold chemistry [7] , [8] , [9] , [10] and many novel body studies [11] . As the mechanisms for trapping ions and atoms differ, so do their energies near the bottom of their respective traps. The combined system, therefore, presents the problem of how the trapped ions and atoms interact with each other and exchange energy and whether the combination is stable. The trap type, energy of the trapped particles, cooling mechanisms and other details impact the manner and rate of energy exchange between ions and atoms. The long range ion–atom potential is of the form −α/ r 4 , where α is the static electric polarizability of the atom and r is the ion–atom separation. The scattering mediated by this potential is the primary channel for the exchange of energy between the ions and the atoms. In the present experiment Rb + (rubidium) ions are confined in a linear Paul trap, which has a trap depth of a few electronvolt (eV). On the other hand the typical temperature of the Rb atoms, which are laser cooled in the magneto-optically trapped (MOT) is of the order of 100 μK (10 −8 eV). This large difference in the energies of the ions and the cold atoms results in the exchange of energy between them, which needs to be understood to exploit the experimental possibilities of the combined system. As Rb + ions have a closed shell electronic configuration, they are not amenable to direct laser cooling. In addition, trapped ions heat [12] due to factors such as trap imperfections, background gas collisions and radiofrequency (RF) heating due to ion–ion repulsion. In this study, collision with cold atoms is the only available cooling channel for Rb + ions. A combined experimental, analytical and numerical approach is attempted here to understand the consequence of mixing optically dark ions and laser-cooled atoms as described below. We first show in general that the elastic collision-mediated cooling between ions and localized cooled atoms, is possible for all ion–atom mass ratios. This is contrary to the general expectation for buffer gas ion cooling [13] , wherein ion cooling should result only for the case when the mass of the ion is much greater than the mass of the atom. The reason for the difference in cooling outcomes is explained within the theoretical framework that applies to both MOT and buffer gas density distributions. For the specific case of Rb + ions and Rb MOT atoms, the role of resonant charge exchange is explored in detail and the mechanism of swap cooling of ions in a single collision is explained. It is numerically demonstrated that ion cooling for equal ion–atom mass ratios is robust for two cases, when only elastic collisions are considered and when elastic and charge exchange collisions are both considered. Experimental studies with this system are then presented, which show that in the limit of long ion–atom hold times the number of trapped ions stabilize, whereas the measured width of the ion distribution continues to shrink. In the absence of the cold atoms the trapped ions evaporate out of the trap rapidly. This loss rate of ions from the trap is used to determine the ion-heating rate. Incorporating the ion-heating rate into our ion-cooling simulation yields ion number stabilization at long hold times, consistent with the experimental observations. A novel technique involving the virial theorem and molecular dynamics (MD) simulation, in conjunction with the experimental data, is used to evaluate the temperature of the optically dark ions in the trap. The arrivial time distribution of the ions on the detector is mapped to the trapped ion temperature. A fall in the temperature is shown, demonstrating the experimental cooling of the ions by the MOT atoms. The combination of ion cooling and constant ion number in the trap demonstrates the intrinsic stability of the ion trap and MOT system. Experimental setup The experimental schematic is illustrated in Fig. 1 . The details of the experimental apparatus [6] are described briefly in the Methods section. The saturated MOT with 2.3(±0.2)×10 6 atoms has a Gaussian density distribution (s.d. ≈ 0.43 mm) and is formed at the centre of the ion trap secular potential (origin). As seen in Fig. 1 , the linear ion trap volume ( v IT ) is much larger than the volume of the cold atoms in the MOT ( v MOT ). The apparatus allows for simultaneous trapping of ions and cold atoms with spatial overlap and to study the evolution of the respective populations for different interaction times. 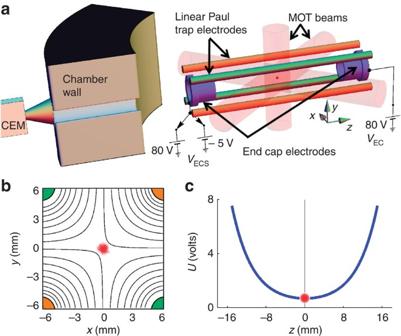Figure 1: The schematic of the experimental setup. The nested MOT in the linear Paul trap with CEM is illustrated in (a). The ion–atom combined trap is constructed, so as to coincide the MOT centre with the minimum of the ion trap secular potential, at the origin. The MOT is formed at the intersection of the six cooling and repumper beams. Ions are created from the excited MOT atoms, by absorption of a photon from a blue light source (not shown). The out of phase oscillating voltage on the quadrupole electrodes, shown in (b) effectsx−ytrapping, whereas a constant end electrode voltageVEC=80 V confines along thezdirection as seen in (c). The approximate size of the MOT is illustrated in red in the cut views of the ion trap potential, demonstrating vMOT≪vIT. The confined ions are detected by a CEM (housed in an evacuated extension to the main chamber), post extraction from the trap, by switchingVECSbetween +80 to −5 V as shown. The port hole in the outer wall of the chamber constitutes a drift region for ToF measurement of the ions extracted. Figure 1: The schematic of the experimental setup. The nested MOT in the linear Paul trap with CEM is illustrated in ( a ). The ion–atom combined trap is constructed, so as to coincide the MOT centre with the minimum of the ion trap secular potential, at the origin. The MOT is formed at the intersection of the six cooling and repumper beams. Ions are created from the excited MOT atoms, by absorption of a photon from a blue light source (not shown). The out of phase oscillating voltage on the quadrupole electrodes, shown in ( b ) effects x − y trapping, whereas a constant end electrode voltage V EC =80 V confines along the z direction as seen in ( c ). The approximate size of the MOT is illustrated in red in the cut views of the ion trap potential, demonstrating v MOT ≪ v IT . The confined ions are detected by a CEM (housed in an evacuated extension to the main chamber), post extraction from the trap, by switching V ECS between +80 to −5 V as shown. The port hole in the outer wall of the chamber constitutes a drift region for ToF measurement of the ions extracted. Full size image Ion cooling mechanism To show that the collisions between the trapped ions and the cold atoms in the MOT leads to cooling of the ions, we closely follow the early, seminal work of Major and Dehmelt [13] . In describing the ion–atom collisions, the MOT atom temperature of ≈100 μK permits us to set the velocity of the atom before a collision, v A =0. If the instantaneous velocity of the ion before a collision is c , its velocity after the collision c ′ is given by where θ c is a unit vector oriented at an angle θ c with respect to c , m I is the ion mass, m A the atom mass and M = m I + m A . θ c corresponds to the angle of deflection of the ion in the centre of mass reference frame. The ion motion can be decomposed into its macromotion and its in-phase micromotion oscillation with the applied electric field [14] . The pre- and post-collision ion velocities then are c = u + v and c ′ = u ′ + v , where u and u ′ are the respective secular velocities, v ∝ E sin(φ RF ), is the micromotion velocity and φ RF is the phase of the electric field E at the instant of collision. The change in ion temperature on undergoing collisions is principally due to a change in its 〈 u 〉, as a collisional change in the position-dependent v results only in a dephasing of the ion's micromotion. So the quantity of interest is 〈 u ′2 − u 2 〉, which gives a measure of the extent of the change in the ion's kinetic energy averaged over long times. Substituting c = u + v and c ′ = u ′ + v in equation (1) and with some regrouping of the terms, we obtain an expression for u ′2 − u 2 as In conventional buffer gas-cooling techniques, a nonreactive buffer gas in thermal equilibrium with a reservoir floods the entire ion trap volume with collisions possible at all parts of an ion's trajectory. But as the ion spends most of its time at the classical turning points of its macromotion, where 〈| u |〉→0 and 〈| v |〉 ≫ 0, most collisions happen there and we can make the approximation This results in the right-hand side of equation (2) being negative for m A ≪ m I, which is a case of ion cooling, positive for m A ≫ m I, which leads to ion heating, and no net change of ion temperature for m A = m I . In our experiment, the cloud of cold atoms acts as the buffer gas and its density distribution is localized around the centre of the ion trap as v MOT ≪ v IT . So the ion–atom collisions happen preferentially at the centre of the trap, which corresponds to the limiting case of 〈| u |〉 ≫ 0 and 〈| v |〉→0. Evaluating equation (2) above in this limit and after carefully taking a time average over φ RF , we obtain the expression for 〈 u ′ 2 − u 2 〉 as, For a given deflection angle, this quantity is negative irrespective of m I / m A and its magnitude is highest for m A = m I . In other words, there is a reduction in the average macromotion energy of the ion in each collision and that the maximum cooling in a collision, for any particular deflection angle, occurs for the equal mass case. This indicates that a spatially compact density distribution of the buffer gas leads to the cooling of the ions. Swap cooling by resonant charge exchange The analysis above is valid for elastic scattering with a fixed scattering angle θ c in the centre of mass frame for any general combination of ion and atom species. For the specific case of Rb + –Rb collisions the resonant charge exchange (RCx) channel [15] , [16] , [17] , [18] is also a dominant channel, which needs to be considered in the collisions between the ions and atoms. In an RCx collision, the valence electron of the atom transfers from the atom to the ion with no other change in the dynamical or internal states of the colliding partners, apart from swapping their respective charge states. For low ion–atom collision energies ( E ) involved in the experiment, the RCx cross section σ cx ∝ 1/ E 1/2 , is comparable to the ion–atom elastic cross section [17] , [19] σ el ∝ 1/ E 1/3 , so both channels participate in ion cooling. At higher energies, the charge exchange, which depends on the molecular state overlap is a very slowly varying function of energy and therefore dominates. In those glancing collisions where RCx occurs, the swapping of the charge state results in an ion almost at rest. This swap cooling occurs preferentially at the ion trap minimum, where the MOT density is maximum. As glancing collisions are overwhelmingly more probable than head-on collisions, the RCx mechanism for transferring energy from ions to atoms can dominate the elastic channel. The difference in the evolution of ion cooling by these two processes in a multiple scattering framework is illustrated by the numerical simulations discussed below. Numerical validation for the collisional cooling of ions Trajectories of 100 noninteracting trapped ions are computed, each undergoing multiple collisions within a Gaussian density distribution (s.d.=0.43 mm) of atoms about the ion trap centre. Elastic [15] , [20] and RCx [21] , [22] collisions are both incorporated in the simulation. The ions are evolved in the experimental potential [6] , from a random initial position distribution, which is much bigger than the extent of the atomic distribution, for elastic only and the elastic with RCx collisions. All collisions are instantaneous and the ion–atom binary interaction potential [20] , [21] determines the specifics of the scattering event. The number of RF cycles between collisions is sampled from a Poisson distribution with a mean of 20 RF cycles and the exact instant of collision within the chosen cycle is randomized uniformly. This procedure ensures the randomness of successive ion–atom collisions, while contracting the time interval over which the ion trajectory needs to be calculated between collisions, allowing the simulation to be experimentally realistic and computationally feasible. Each collision occurs with an impact parameter b chosen from a probability distribution p b ( b ) ∝ b such that 0< b < b max where b max corresponds to a scattering angle θ c >60 microradian. The elastic collisions can result in simple angular deflections that do not cross the angular momentum barrier or the more complicated inspiralling orbital motion depending upon whether the impact parameter is greater or lesser than a certain critical impact parameter b cel , respectively. The cross-section σ L =π b 2 cel corresponding to this impact parameter is often referred to as the Langevin cross-section and the cross-section for charge-exchange tends to this value at low energies. At higher energies, the charge exchange is active outside the centrifugal barrier and we can define a critical impact parameter for charge exchange b cx such that when b ≤ b cx , the average probability for RCx is 1/2 and for b > b cx the probability of RCx rapidly falls to zero. The value of b cx is determined from the Rb + –Rb molecular potential [21] , [22] . The two critical impact parameters b cel and b cx are plotted in Fig. 2 as a function of the approach velocity for the 85 Rb system. The collision results in the change of ion velocity from c → c ′ . The kinematics of the collision are computed following the treatment in McDaniel [15] . 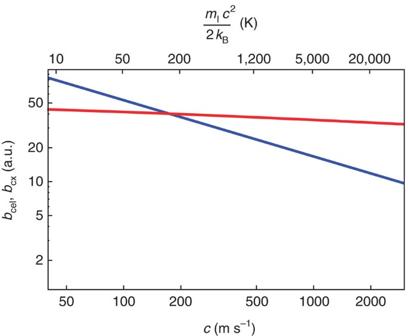Figure 2: Critical impact parameters for elastic and charge exchange collisions as a function of ion velocity. The plot of the critical impact parameters in atomic units (a.u.), for elastic collisionsbcel(blue) and RCxbcx(red) as a function of the approach velocity of the ion and the atom is shown in a log-log scale. At high values of the collision energy, the value ofbcxis substantially higher than that ofbceland charge exchange happens way above the centrifugal barrier. In this regime, a fast ion at a high impact parameter can exchange its charge state with an atom at rest resulting in a slow ion and a fast atom. In effect, the ion and the atom swap their dynamical states and a cold ion can result from a single collision at the ion trap centre. The top axis denotes the velocity equivalent temperature to make contact with the results described below. Figure 2: Critical impact parameters for elastic and charge exchange collisions as a function of ion velocity. The plot of the critical impact parameters in atomic units (a.u. ), for elastic collisions b cel (blue) and RCx b cx (red) as a function of the approach velocity of the ion and the atom is shown in a log-log scale. At high values of the collision energy, the value of b cx is substantially higher than that of b cel and charge exchange happens way above the centrifugal barrier. In this regime, a fast ion at a high impact parameter can exchange its charge state with an atom at rest resulting in a slow ion and a fast atom. In effect, the ion and the atom swap their dynamical states and a cold ion can result from a single collision at the ion trap centre. The top axis denotes the velocity equivalent temperature to make contact with the results described below. Full size image The mean ion kinetic energy (〈 T K 〉) for the cases where only the elastic channel is active and both elastic and RCx channels are active is shown in Fig. 3 . Ion cooling is clear from the reduction of mean kinetic energy per ion of the noninteracting ions in the trap with time. The ions cool much faster when the RCx channel is active along with the elastic one. The initial spatial distribution of the ions is taken to be much bigger than the FWHM of the atom density distribution to emphasize the role of compactness in the distribution of atoms for ion cooling. 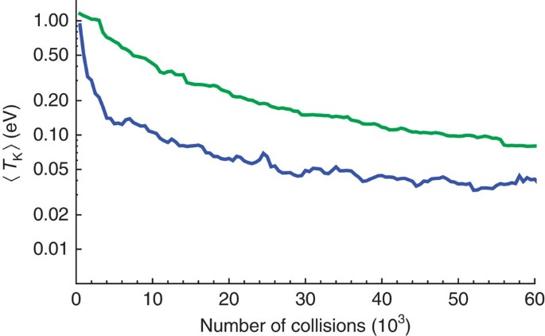Figure 3: Numerical results for collisional cooling of ions. The fall in average ion kinetic energy as a function of the total number of collision events (which corresponds directly to evolution time) for the simulation of 100 independent ions with the localized atoms. Here the green and blue lines represent elastic and elastic+RCx collisions, respectively. In both cases 〈TK〉 decreases with collision number. However, we note that for the elastic+RCx collision, the reduction in 〈TK〉 requires fewer collisions when the ions are more energetic. Figure 3: Numerical results for collisional cooling of ions. The fall in average ion kinetic energy as a function of the total number of collision events (which corresponds directly to evolution time) for the simulation of 100 independent ions with the localized atoms. Here the green and blue lines represent elastic and elastic+RCx collisions, respectively. In both cases 〈 T K 〉 decreases with collision number. However, we note that for the elastic+RCx collision, the reduction in 〈 T K 〉 requires fewer collisions when the ions are more energetic. Full size image Experimental results Our hypothesis for ion cooling is experimentally implemented and verified by measuring the evolution of the ion population in the trap as follows. The Rb dispenser and the quadrupolar magnetic field for the MOT are kept ON throughout the measurement. Initially, the MOT is loaded for τ ml =40 s until saturation, during which the ion trap RF field is kept OFF. Once the MOT is saturated, the ion trap's RF field is switched ON and a small fraction of the atoms in the MOT are ionized by pulsing ON the ionizing blue light for τ il =1 s to load the ion trap. At the end of the ion-loading interval, the cold atoms can be retained in the trap or can be ejected within a few milliseconds by simultaneously switching OFF the cooling and repumper lasers with a mechanical shutter. The ions are trapped for a further hold time, τ ih , either without MOT atoms or with MOT atoms, following which they are extracted onto the channel electron multiplier (CEM) by switching V ECS . The ion count detected on the CEM is measured as a function of τ ih separately for the two cases. The CEM ion counts versus τ ih is plotted in Fig. 4a and the FWHM of the ion arrival time-of-flight (ToF) distribution in Fig. 4b . When the MOT is switched off, all the ions exit the trap by τ ih ≈ 15 s and the ToF FWHM increases rapidly. The rapid loss of ions from the trap, and the increase in the width of the arrival time distribution are shown in the insets of Fig. 4a,b , respectively. On the other hand, when the ions are held in the presence of the MOT, for τ ih ≥ 1 s, the ion loss rate from the trap drops and so does the FWHM of the ion ToF distribution. Beyond τ ih ≥ 2 min, the number of trapped ions stabilizes to a constant value, wheras the width of the ToF distribution decreases, indicating that ion cooling is still under way. We therefore conclude that a number equilibrium between daughter ions and laser-cooled parent atoms is achieved and a thermally stable equilibrium exists within experimental means. 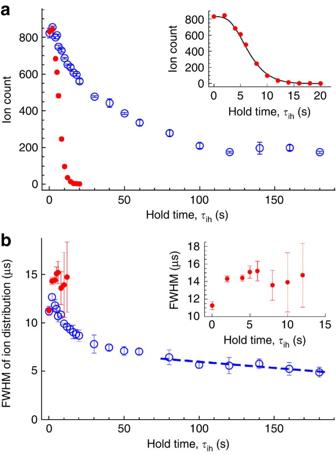Figure 4: Experimental demonstration of ion cooling. Evolution of trapped ion population and distribution is experimentally determined when the ions are held in the trap without MOT atoms (red filled circles) and with MOT atoms (blue empty circles). (a) Plots the number of Rb+ion counts as a function ofτih. Without a MOT, the ions exit the trap rapidly, whereas with cold atoms the ion loss is much slower and a stable number of ions (187±9) is trapped without detectable loss beyondτih≥2 min. The inset in (a) shows the detail of the ion loss (red circles) when the ions are held without the MOT atoms. This ions loss is fitted with a function (black solid line) obtained by the Monte–Carlo model described in the text. (b) Illustrates the variation of the FWHM of the ion ToF distribution againstτih. In the absence of the MOT atoms, the FWHM increases in time as the trap empties out, the detail of which is shown in the inset. In contrast, when ions are held with the MOT atoms, a systematic decrease in the ion ToF distribution is seen, consistent with ion cooling. Forτih≥2 min, when the trapped ion number has stabilized, the ToF width is still decreasing indicating continued ion cooling, as illustrated by a least square fit to the last six data points. The statistical s.d.e. bars are shown. Figure 4: Experimental demonstration of ion cooling. Evolution of trapped ion population and distribution is experimentally determined when the ions are held in the trap without MOT atoms (red filled circles) and with MOT atoms (blue empty circles). ( a ) Plots the number of Rb + ion counts as a function of τ ih . Without a MOT, the ions exit the trap rapidly, whereas with cold atoms the ion loss is much slower and a stable number of ions (187±9) is trapped without detectable loss beyond τ ih ≥2 min. The inset in ( a ) shows the detail of the ion loss (red circles) when the ions are held without the MOT atoms. This ions loss is fitted with a function (black solid line) obtained by the Monte–Carlo model described in the text. ( b ) Illustrates the variation of the FWHM of the ion ToF distribution against τ ih . In the absence of the MOT atoms, the FWHM increases in time as the trap empties out, the detail of which is shown in the inset. In contrast, when ions are held with the MOT atoms, a systematic decrease in the ion ToF distribution is seen, consistent with ion cooling. For τ ih ≥2 min, when the trapped ion number has stabilized, the ToF width is still decreasing indicating continued ion cooling, as illustrated by a least square fit to the last six data points. The statistical s.d.e. bars are shown. Full size image Determination of the trapped ion-heating rate The analysis of the ion–atom heat exchange first requires the ion heating rate in the absence of the MOT atoms. This is computed from the experimental data using a Monte–Carlo calculation for a noninteracting distribution of ions, to model the loss of ions from the trap in the absence of atoms. We assume a homogeneous exponential antidamping factor Γ to collectively represent the different heating mechanisms of the ions. This is a reasonable approximation when there is no cooling mechanism and the ion cloud is dilute, implying that ion trajectories are largely independent of each other. An ion with initial position ( x i , y i , z i ) sampled from the MOT density distribution, evolves in the ion trap potential with the antidamping factor Γ. The ion exits the ion trap at time t ej , when it's kinetic energy exceeds E ej , where the relation between t ej and E ej (details in the Methods section) is written as, where x 0 = x i /(1+ q /2), y 0 = y i /(1− q /2) and z 0 = z i , Ω is the drive frequency, q is the Mathieu stability parameter and ω r and ω z are the secular oscillation frequencies in the radial and axial directions, respectively. E ej is the maximum kinetic energy including the micromotion energy that the ion can possess and still remain in the trap. The time of ejection t ej of the ion for each initial position is determined using equation (4). The cumulative probability distribution for t ej gives the fraction of ions ejected from the trap at a certain time and from this the fraction of ions remaining in the trap, at different times is determined. The model curve is compared with the measured data of Fig. 4 in the absence of MOT atoms for different values of Γ and E ej and the pair of (Γ, E ej ) for which the χ 2 of the fit is minimized is chosen. The model and the data are shown in the inset of Fig. 4a for Γ=5.7×10 −24 kg s −1 and E ej =2.83 eV. This value for E ej corresponds to a secular motion energy of 0.8 eV. Ion number stabilization with ion heating Having determined the experimental ion-heating rate, it is important to verify that the earlier ion-cooling simulations still predict ion cooling and ion number stabilization. To qualitatively study the stability of ions in the presence of the atoms, multiple-collision numerical simulations for 100 noninteracting ions are performed with the antidamping factor Γ included. As the rate of ion heating is expected to vary with varying ion population and density in the presence of the atoms a constant Γ cannot be expected to replicate the quantitative features. However, in the absence of knowledge for the time dependence of Γ we take Γ=5.7×10 −24 kg s −1 throughout. The initial ion positions are generated from the density distribution of the MOT and the impact parameter b is computed as before. To calculate over time scales comparable to the experiment, the average macromotion speed 〈 u 〉 of the ion is computed over the average atomic density n̄ that it passes through, to determine the time interval before the next collision as where σ s =π b 2 max is the cross-section corresponding to the maximum sampled impact parameter. The calculated ion trajectories are then analysed to determine the fraction of the ion population remaining in the trap as a function of time for τ ih =50 s. The elastic and the RCx channels for ions and atoms in the ground state are incorporated as described earlier. The collisions in the excited state and the stochastic nature of the excitation and de-excitation of atoms are not considered. The result of this simulation, shown in Fig. 5 , exhibits a qualitative correspondence to the blue trace of Fig. 4a and confirms the ion number stabilization that accompanies ion cooling as a function of ion hold times. 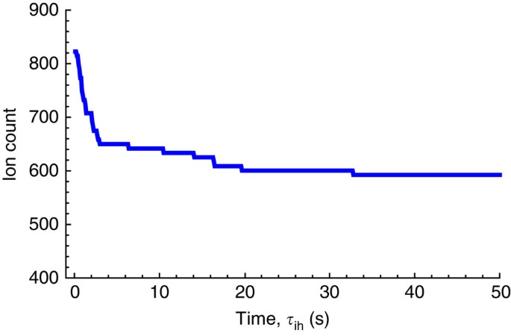Figure 5: Numerical study of ion number stabilization with cooling and heating. The evolution of the ion population with hold timeτihas computed from the multiple collision simulations in the presence of the exponential antidamping factor. The simulations give the fraction of the initial ion population, which is scaled to the experimentally observed ion population atτih=0. We note that this is qualitatively similar to the sequence of blue circles ofFig. 4a. Figure 5: Numerical study of ion number stabilization with cooling and heating. The evolution of the ion population with hold time τ ih as computed from the multiple collision simulations in the presence of the exponential antidamping factor. The simulations give the fraction of the initial ion population, which is scaled to the experimentally observed ion population at τ ih =0. We note that this is qualitatively similar to the sequence of blue circles of Fig. 4a . Full size image Ion temperature determination Given that the constant number of trapped ions for τ ih >2 min ( Fig. 4a ) and a systematic decrease in the arrival time widths ( Fig. 4b ), the temperature at any hold time is evaluated as follows. An ion distribution, consistent with a given temperature value, is evolved within a numerically generated potential for the ion trap system that includes the CEM, using an interacting ion MD [24] simulation. Interacting ion simulation is needed here to accurately account for lensing effects in the extraction and detection processes. The ions are subjected to the transient extraction potential of the ion trap and their arrival times at the detector's position are analysed. The response function for the detector circuit is convolved onto the extracted ion distribution so that the experiment is mimicked with precision by the simulation. The positions and velocities of trapped ions, consistent with a specific temperature are generated using the virial theorem [23] . To use this we assume that the ion–ion and ion–atom interactions are negligible. This is reasonable because the ion–ion collisions are occasional and the ion–atom collisions are rare within a single macromotion cycle, which is a natural time to take an average over. The surviving trap potential term after time averaging over the macromotion cycle can be substituted by the corresponding harmonic secular potential ( U ext ) and the virial equation for the present problem reduces to 〈 T K 〉 ≈ 〈 U ext 〉. This equation determines the relation between the spatial and velocity distributions of ions at temperature T in the trap. The variances of the position and velocity distributions consistent with temperature T is now given by where the ω i are the macromotion frequencies, k B is the Boltzmann constant and m I is the mass of the ion. Multiple ion ensembles are generated using the above distribution widths for different temperatures. Each ensemble is evolved for a few macromotion cycles and extracted in the interacting ion MD simulation. The arrival time distribution recorded is plotted against the temperature in Fig. 6 , which relates the experimentally measured width of the ToF distribution in Fig. 4b to the temperature of the ion cloud. From this analysis we evaluate the temperature for the trapped ions as ≈30 K at τ ih =180 s. The above temperature value represents an upper bound for the ion system so held. The ion system is capable of lower temperatures; however, our ability to determine the ion temperature significantly below this value, by the method described above, is limited. This is because at lower temperatures, for a fixed ion number, the ion density increases. The resulting increase in the ion–ion interaction then invalidates the approximate form of the virial theorem described above, and therefore compromises further temperature measurements. In addition, at very low ion temperatures the sensitivity of this method drops as the ion ToF width varies marginally with temperature. Nevertheless, over the range of the present experiment, this analysis is robust and reliable and therefore suitable for the temperature measurement of trapped, optically dark ions. 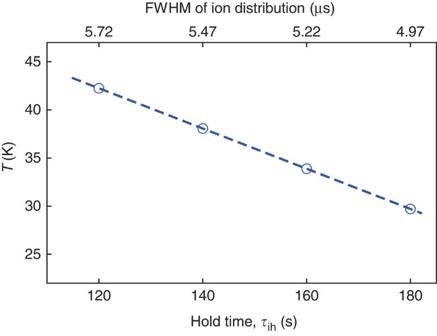Figure 6: Ion temperature determination. The trapped ion ensemble temperature is determined for the duration when the ion number has stabilized, that is for 2≤τih≤ 3 min. For this duration the temperature fit to the trapped ions as obtained from MD simulations (dashed line) is plotted as a function of trap hold time. The corresponding experimental ToF width of the extracted ions is marked on the top axis. The open circles represent the hold times at which the experimental measurements were made. Figure 6: Ion temperature determination. The trapped ion ensemble temperature is determined for the duration when the ion number has stabilized, that is for 2≤ τ ih ≤ 3 min. For this duration the temperature fit to the trapped ions as obtained from MD simulations (dashed line) is plotted as a function of trap hold time. The corresponding experimental ToF width of the extracted ions is marked on the top axis. The open circles represent the hold times at which the experimental measurements were made. Full size image In the above study of ion-cooling mechanisms we have exclusively focussed on the binary ion–atom interaction. Within this restriction we demonstrate that the ions are effectively cooled by collision with the localized, cold MOT atoms. It is the continuous atom cooling, which indirectly bleeds away energy from the trapped ions, and the constant number of atoms in the reservoir (MOT) that has the capacity to cool the ions. Without these two features simultaneously in place, the trapped ions will empty the atom trap very quickly, because of ion heating by various mechanisms and the relatively strong −α/ r 4 ion–atom interaction potential. The effect of ion–ion interactions on the cooling and the stabilization of the ion numbers has not been numerically addressed as we are in the dilute ion limit. However, we have incorporated the Coulomb repulsion of the ions for the MD simulation used in the evaluation of the ion temperature. The existence of ground and excited-state populations within the cold atoms, with different polarizabilities, has been ignored in the discussions. Although these have an important role in the determination of the final state of the system, these details are not of primary relevance to the binary collisional cooling principle demonstrated here. Even in the charge exchange channel, there is no contribution of energy to the collision from internal-state changes. Therefore, the parent–daughter atom–ion system demonstrates ion cooling and long-term stability unequivocally. In conclusion, we have shown that localized parent atom–daughter ion collisions allow a viable ion cooling technique. The cooling is understood from simple theoretical considerations for elastic collisions. It is numerically demonstrated that RCx accelerates the collisional ion cooling process. The experimental data illustrates that in the limit of long hold times, the number of trapped ions becomes constant, whereas the spread in the ion arrival times at the detector continues to shrink, implying continued cooling. The stabilization of trapped ion numbers is demonstrated numerically in a multiple ion–atom scattering simulation, where ion–ion interactions are ignored, but the experimentally determined ion-heating rate is incorporated. The temperature of the trapped ions, once the ion population has stabilized is determined using a combination of the virial theorem and a fully interacting ion MD evolution and detection of the ion ensemble. The ion temperatures and cooling rates are in line with the experimental expectations and further cooling is given. We therefore conclude that a stable ion–atom ensemble is experimentally possible. The direct consequence of the cooling and stability demonstrated here then allows various mixtures of ions and atoms to simultaneously co-exist, whether the ions are laser coolable or not. These results lead to intriguing questions for future study such as, what is the equilibrium state and configuration of the cooled ion–atom system? How are collective oscillations of the ions damped in this RCx active system? Most significantly, the cold ion–atom ensemble that we have studied is a self-stabilizing system and sets the stage for ion-involved production of cold molecules and generalization to studies with multiple species. Experimental construction and operation The Rb MOT is vapour loaded by heating a Rb source. The MOT has six independent laser beams of 1 cm diameter and a gradient magnetic field of 12 Gauss cm −1 . Measurements on the cold atoms are made by fluorescence detection and optical imaging. The Rb + ions are created with negligible recoil from the trapped MOT atoms by two photon ionization, where one photon is available from the cooling laser itself. The second photon (456 nm), is emitted by a light-emitting diode, which is switched on to create ions from the excited MOT atoms. The ion trap is a linear Paul trap with hollow cylindrical end caps as shown in Fig. 1 . A sinusoidal voltage of amplitude V RF =91 V, frequency Ω=2π × 600 kHz with 180° phase difference between adjacent rods is applied for x–y confinement. Confinement in z is effected by a DC voltage V EC =80 V applied to end electrodes along the z axis. These ions are destructively detected by sweeping out the trapped ions through the hollow-end electrode and a drift region, onto a CEM, by switching the voltage, V ECS from 80 V →−5 V. The CEM and a preamplifier assembly together convert the incident extracted ions from the trap to a proportional voltage signal. Energy evolution of an antidamped ion in a linear Paul trap Consider an ion initially at a point ( x i , y i , z i ) in a linear Paul trap operating at a RF voltage of amplitude V RF and frequency Ω. The Mathieu stability parameter in the radial direction is where r 0 is a geometrical constant of the trap. Let the secular frequencies in the radial and axial direction be ω r and ω z , respectively. For q<1, the ion's trajectory in the presence of an antidamping factor Γ is given by The energy of the ion rapidly oscillates between zero and a maximum value and this maximum value changes over time under the influence of Γ. The time-derivatives of equation (5) give the corresponding instantaneous velocities. Squaring each velocity, we substitute the quadratic oscillatory terms with the corresponding maximum values and neglect the linear oscillatory terms. The remaining time dependence is in the form of the exponential antidamping factor. The maximum kinetic energy contributions from each direction are obtained as Summing these, the evolution of the maximum total kinetic energy, including the micromotion is subsequently obtained as When q is not so small compared with unity, the expression for the ion's trajectory is not well represented by equation (5). But the expression for the energy envelope equation (7) still remains a good approximation. How to cite this article: Ravi K. et al . Cooling and stabilization by collisions in a mixed ion–atom system. Nat. Commun. 3:1126 doi: 10.1038/ncomms2131 (2012).